Stiffening hydrogels to probe short- and long-term cellular responses to dynamic mechanics Biological processes are dynamic in nature, and growing evidence suggests that matrix stiffening is particularly decisive during development, wound healing and disease; yet, nearly all in vitro models are static. Here we introduce a step-wise approach, addition then light-mediated crosslinking, to fabricate hydrogels that stiffen (for example, ~3–30 kPa) in the presence of cells, and investigated the short-term (minutes-to-hours) and long-term (days-to-weeks) cell response to dynamic stiffening. When substrates are stiffened, adhered human mesenchymal stem cells increase their area from ~500 to 3,000 μm 2 and exhibit greater traction from ~1 to 10 kPa over a timescale of hours. For longer cultures up to 14 days, human mesenchymal stem cells selectively differentiate based on the period of culture, before or after stiffening, such that adipogenic differentiation is favoured for later stiffening, whereas osteogenic differentiation is favoured for earlier stiffening. Cells sense their surrounding matrix mechanics by pulling and pushing it, and in response, generate biochemical activity through a process known as mechanotransduction [1] , [2] . In the last decade, matrix stiffness alone has been implicated in regulating cellular functions, such as contraction [3] , [4] , migration [5] , [6] , proliferation [7] , [8] and differentiation [9] , [10] . With this in mind, a variety of natural (for example, gelatin, collagen) and synthetic (for example, polyacrylamide) polymer systems were used in vitro to mimic the elasticity of native tissues, which varies significantly throughout the body (for example, brain: ~0.2–1 kPa (refs 11 , 12 , 13 ), muscle: ~10 kPa (ref. 10 ), osteoid: ~30–45 kPa (ref. 14 )). Despite helping to develop this important field and gather valuable information, these substrates are primarily static and lack the dynamic nature that is observed during many cellular processes (for example, development, fibrosis, cancer). Thus, it is of great interest to temporally manipulate matrix elasticity in vitro to better understand and develop strategies to control these biological processes. In this regard, biodegradable polymers can be considered as early examples of dynamic systems, where the material mechanics gradually decrease with time via hydrolysis or enzymatic remodelling [15] . More recently, Anseth and colleagues [16] reported on photocleavable polyethylene glycol-based hydrogels, where crosslinking can be decreased both temporally and spatially with light exposure. However, matrix stiffening is more relevant for many biological events, including tissue development, wound healing and disease progression, such as fibrosis and tumour formation. For instance, fibrous scar tissue that develops after myocardial infarction is much stiffer than normal myocardium [17] , [18] , [19] , and mesenchymal stem cells (MSCs) differentiate down an osteogenic lineage and produce markers of bone when injected into infarct tissue in mice [20] . Recent evidence also suggests that matrix stiffening, which is generally regarded as an outcome of disease, may be a contributing factor in disease development. Liu et al . [21] reported that matrix stiffening suppresses cyclooxygenase-2 expression and prostaglandin E2 during fibrosis. Similarly, Levental et al . [22] observed that matrix stiffening induced tumour progression by enhancing integrin signalling. With these examples in mind, cell culture systems with user-defined temporal control of stiffening are essential for fundamental investigation of these processes. Despite this interest, there are only a few examples of systems in which stiffness can be dynamically controlled, none without their limitations. For example, Gillette et al . [23] reported collagen–alginate composite hydrogels, where mechanics are altered with the introduction of divalent cations, yet calcium may alter cell signalling, and the long-term stability of these gels is limited; external stimuli such as pH [24] and temperature [25] , [26] can be used to alter matrix stiffness, but only with large volumetric and hydrophobicity changes; free DNA was used to dynamically control the mechanics of DNA hybrid hydrogels [27] ; however, slow reaction kinetics (vary from 4 h to 1 day) [28] , [29] , [30] , homogeneity through the sample owing to retarded diffusion [31] , significant changes in the net charge of the hydrogel (free DNA is highly negatively charged) [30] , [31] , lack of information on long-term (>7 days) stability of the gels in culture condition, and possible problems with cellular compatibility (the similarity of the DNA sequence to the genome of the specific cell type used) [28] , [32] are some of their limitations. Here we develop and implement a stiffening hydrogel system that provides fast dynamic changes, long-term stability and structural uniformity. By using a model system that permits osteoblast (bone) and adipocyte (fat) differentiation in a bipotential media, we investigate the immediate and long-term human MSC (hMSC) response to substrate stiffening from soft (~3 kPa) to stiff (~30 kPa) in terms of spreading, traction forces (via dynamic traction-force microscopy (TFM)), motility, proliferation and differentiation. We report that hMSCs respond to stiffening immediately with increases in cell area, traction forces and motility, which equilibrate within 2–4 h, and that long-term proliferation and hMSC-fate decisions are dependent on timing of the stiffening. Sequential crosslinking and characterisation In this work, we used hyaluronic acid (HA), a linear polysaccharide that is composed of alternating D -glucuronic acid and N -acetyl- D -glucosamine, as the primary structural unit, because it is a natural component of the extracellular matrix and is involved in many biological processes [33] , [34] . HA may be chemically modified in a variety of ways to form hydrogels with tuneable properties (for example, hydrophobicity, degradation) towards the development of biomaterials for tissue engineering and regenerative medicine [34] , [35] , [36] , [37] . Although sequential crosslinking was previously employed to spatially control hydrogel mechanics without cells present, here, for the first time, we report sequential crosslinking as a route for in situ hydrogel stiffening in the presence of cells ( Fig. 1a ). For this purpose, HA macromers were functionalised with methacrylates via a simple reaction of HA with methacrylic anhydride (MA; Supplementary Fig. S1 ), because methacrylates react with both thiols and radicals for crosslinking. First, hydrogels with uniform mechanical properties were obtained via a Michael-type addition reaction when dithiothreitol (DTT) is introduced into a methacrylated HA (MeHA) solution in triethanolamine buffer, via reaction between some fraction of the methacrylates with the thiols on the DTT. During this initial gelation, the amount of methacrylate groups involved in the crosslinking reaction can be tuned by the concentration of DTT. Next, this initial hydrogel could be further stiffened within minutes by radical polymerisation of the remaining methacrylate groups, at a user-defined time, when the hydrogel is swollen with a photoinitiator (Irgacure 2959 (I2959)) and exposed to ultraviolet light. We used a highly modified MeHA ( Supplementary Fig. S1 ) at a concentration of 3 wt% for all studies and tuned the mechanics through the amount of DTT introduced, and the presence and timing of ultraviolet light exposure. For all studies, the MeHA was modified with an adhesive peptide (arginine–glycine–aspartic acid, RGD), such that the final concentration of this ligand was 1 mM. 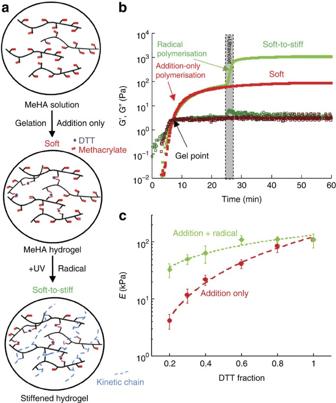Figure 1: Sequential crosslinking approach. (a) Schematic of MeHA crosslinking process. (b) Rheology profiles showing hydrogel formation via addition reaction only (soft, red) and stiffened hydrogel, addition reaction followed by radical polymerisation (soft to stiff, green). Storage modulus (G′) and loss modulus (G′′) are indicated by solid and open labels, respectively. (c) Atomic force microscopy measurement of Young's moduli (E) of MeHA substrates for addition-only polymerisation (red) with varying DTT concentration (at pH 10) and for stiffened substrates (green). Error bars represent s.d. (ten random measurements for each sample withn=3). Figure 1: Sequential crosslinking approach. ( a ) Schematic of MeHA crosslinking process. ( b ) Rheology profiles showing hydrogel formation via addition reaction only (soft, red) and stiffened hydrogel, addition reaction followed by radical polymerisation (soft to stiff, green). Storage modulus (G′) and loss modulus (G′′) are indicated by solid and open labels, respectively. ( c ) Atomic force microscopy measurement of Young's moduli ( E ) of MeHA substrates for addition-only polymerisation (red) with varying DTT concentration (at pH 10) and for stiffened substrates (green). Error bars represent s.d. (ten random measurements for each sample with n =3). Full size image The evolution of network formation during addition-only and sequential crosslinking was monitored by dynamic time-sweep rheological experiments ( Fig. 1b ). For a system using 20% DTT, the initial gelation time (indicated by gel point when the storage modulus ( G′ ) is equal to loss modulus ( G′′ )) occurred within ~6 min, and G′ plateaued within 20 min, indicating complete gelation for addition-only polymerisation. Much stiffer gels formed in shorter times with increasing DTT concentration ( Supplementary Fig. S2 ). A sharp increase in G′ was observed when the addition-only hydrogel was exposed to ultraviolet light for 2 min after ~25 min ( Fig. 1b , shaded area), confirming the radical polymerisation and ability to increase hydrogel mechanics. It is also important to note the fast kinetics of the radical polymerisation, which begins immediately with light exposure and plateaus immediately after light removal. Also, it is noted that the final hydrogel mechanics can be tuned by ultraviolet exposure time ( Supplementary Fig. S2 ). It is also possible to gradually increase the substrate stiffness through multiple ultraviolet exposures ( Supplementary Fig. S2 ). Atomic force microscopy was used to characterise the elastic moduli of the hydrogel substrates ( Fig. 1c ). By simply varying the DTT concentration in the initial MeHA solution, a wide range of substrate mechanics from ~3 to ~100 kPa were observed for the addition-only polymerisation, which were further stiffened through incubation with photoinitiator and 2 min of light exposure, and dependent on the consumption of methacrylates during the first step. Short-term hMSC response to temporal stiffening As stated above, many cell types are responsive to the mechanical properties of their substrate, including towards their spreading behaviour [14] , [38] . Thus, as expected, hMSCs cultured on addition-only hydrogel substrates for 1 day spread in a manner that was dependent on the substrate stiffness ( Supplementary Fig. S3 ), such that the cell area distribution became wider and shifted to higher values with increasing stiffness. Specifically, hMSCs were rounded and less spread with a very narrow distribution of cell area on ~3 kPa substrates, whereas hMSCs spread to a greater extent and possessed organised stress fibres for ~100 kPa substrates. The mean values of cell area ( Ã ) for hMSCs were ~500, 2,500, 5,000 and 7,500 μm 2 for ~3, 20, 40 and 100 kPa substrates, respectively. To investigate the short- and long-term cellular response to substrate stiffening, we used a stiffening substrate that transitioned from ~3 (addition-only, soft) to ~30 kPa (stiffened, soft to stiff) as a model system. For the in situ stiffening system, hMSCs were seeded onto the soft substrate and cultured for various periods; a solution of the I2959 photoinitiator in media was then introduced for 30 min, and the samples were exposed to ultraviolet light for 2 min to stiffen the substrates while the cells were present. To assess the effects of I2959, ultraviolet exposure and their combination, a detailed viability study was performed, including mitochondrial activity and membrane permeability, as well as potential DNA damage via p53 immunostaining analysis ( Supplementary Fig. S4 ). No detrimental effects on hMSC behaviour were observed for our specific experimental parameters with any of these outcomes, providing evidence of negligible damage to the cells during the stiffening process. After 1 day of culture in growth media, hMSCs remained rounded with diffuse F-actin staining on soft substrates, whereas hMSCs spread much greater and possessed strong actin fibres on stiff substrates, which remained similar for both substrates at day 2 ( Fig. 2a ). The rounded morphology of hMSCs on the soft substrate at day 1 changed significantly at day 2 to a spread morphology similar to that of hMSCs on the stiff substrate, in response to substrate stiffening at day 1 ( Fig. 2a ). The distribution of cell areas for hMSCs on soft substrates ( Ã ~500 μm 2 ) became much wider and shifted to much higher values ( Ã ~3,000 μm 2 ), almost identical to that of hMSCs on stiff substrates at day 2 after stiffening at day 1 ( Fig. 2b ). To investigate the immediate response to stiffening, we collected time-lapse images of the cells starting before stiffening. Time-lapse images of hMSCs over a 16-h period on soft, stiff and stiffened (soft to stiff at day 1) substrates illustrate an increase in mean cell area from ~400 to ~1,500 μm 2 within 4 h immediately on stiffened substrates, and little change in cell area on soft (~400 μm 2 ) and stiff (~1,500 μm 2 ) substrates during this period ( Fig. 2c ). With respect to focal adhesions, hMSCs on soft substrates showed diffuse vinculin (focal adhesion marker) staining, whereas mature vinculin patches were observed for hMSCs on stiff substrates at day 1 and day 2, and on stiffened substrates at day 2 ( Supplementary Fig. S5 ). To determine the effect of ligand (RGD) concentration on hMSC spreading, soft substrates with a wide range of RGD concentration (from 0 to 2 mM) were fabricated ( Supplementary Fig. S6 ). No significant changes in cell morphology and spreading were observed before and after stiffening, except for the case without RGD, in which we observed little cell adhesion. 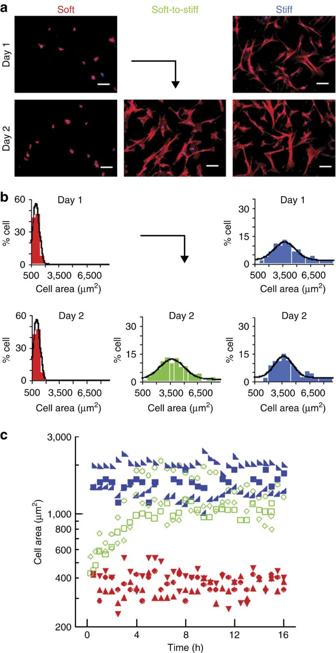Figure 2: Effect ofin situstiffening on cell spreading. (a) Fluorescent images of hMSCs cultured on MeHA substrates for 1 and 2 days with indicated stiffness (soft, 3 kPa; stiff, 30 kPa; soft-to-stiff, 3–30 kPa).In situstiffening of soft gels is performed at day 1. Scale bars are 100 μm. (b) Distributions of cell areas (n>200) when cultured on substrates with corresponding stiffness conditions in (a). (c) Evolution of cell area changes for hMSCs in real-time response to stiffening (green). Soft substrate is stiffened att=0 h. The cell area of hMSCs on soft (red) and stiff (blue) substrates are also included as controls and show little change with culture time. Each data set (n=3) is for an individual cell for 16 h. Figure 2: Effect of in situ stiffening on cell spreading. ( a ) Fluorescent images of hMSCs cultured on MeHA substrates for 1 and 2 days with indicated stiffness (soft, 3 kPa; stiff, 30 kPa; soft-to-stiff, 3–30 kPa). In situ stiffening of soft gels is performed at day 1. Scale bars are 100 μm. ( b ) Distributions of cell areas (n>200) when cultured on substrates with corresponding stiffness conditions in ( a ). ( c ) Evolution of cell area changes for hMSCs in real-time response to stiffening (green). Soft substrate is stiffened at t =0 h. The cell area of hMSCs on soft (red) and stiff (blue) substrates are also included as controls and show little change with culture time. Each data set ( n =3) is for an individual cell for 16 h. Full size image TFM was used here to investigate the immediate and short-term dynamic response to substrate stiffening ( Supplementary Fig. S7 ). Specifically, hMSCs were cultured on soft substrates for 1 day, and cells were tracked immediately after substrate stiffening for 15 h and compared with uniform culture on soft or stiff substrates. No significant changes in average traction forces by hMSCs were observed on soft and stiff substrates during this period ( Fig. 3a,b ). However, in response to substrate stiffening, the average traction of hMSCs increased significantly from ~1 to 10 kPa within ~4 h, and then plateaued at a level similar to hMSCs cultured on stiff substrates. 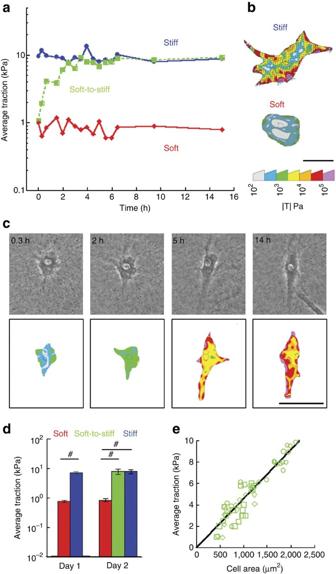Figure 3: Effect ofin situstiffening on cell traction forces. (a) Real-time change in average traction force exerted by representative hMSCs cultured on stiff (blue), soft (red) andin situ-stiffened (soft to stiff, green) hydrogels. (b) Colour traction maps of representative hMSCs on stiff and soft MeHA hydrogels. The pseudocolour bar indicates the spatial traction forces, |T|, in Pa. Scale bar is 25 μm. (c) Time-lapse phase-contrast images and corresponding traction stress maps of a representative cell showing the real-time response toin situstiffening (same cell). Colour map indicates the magnitude of the cellular traction stresses. Scale bar is 50 μm. (d) Average cellular traction force per cell area for hMSCs cultured on soft (3 kPa) and stiff (30 kPa) hydrogels for 1 day. Error bars represent s.e. (n=20). #denotesP<0.001. (e) Average cellular traction plotted against corresponding cell area over a 14 h period, immediately afterin situstiffening. Each data set represents an individual cell (n=3). Linear fit is plotted as solid line (slope=0.046). Time-lapse phase-contrast images of a typical cell on a stiffened substrate accompanied with corresponding colour traction maps are provided in Figure 3c . When quantified over a range of cells, the average traction on soft and stiff substrates were significantly different, ~1 kPa for soft and ~10 kPa for stiff, but there was no statistical difference for either formulation between day 1 and day 2 ( Fig. 3d ). Also, there was no statistical difference for average traction forces between hMSCs on the stiff substrates and on the stiffened substrate at day 2. Regarding the temporal nature of the cells after stiffening, there was a linear correlation between the mean magnitude of traction exerted by a cell and the increase in cell spread area, over the 4-h period following the stiffening process ( Fig. 3e ). This is in agreement with the behaviour observed for cells during spreading after seeding onto a substrate [39] . Cell motility was also affected by substrate mechanics ( Supplementary Fig. S8 ) such that the mean velocity and mean accumulated distance of hMSCs on soft substrates were significantly lower than that of hMSCs on stiff substrates. For hMSCs on stiffened substrates, the average cell motility was significantly lower than that of the cells on stiff substrates for 16 h immediately after stiffening, indicating little motility during the spreading process ( Supplementary Movies 1 , 2 , 3 ). Figure 3: Effect of in situ stiffening on cell traction forces. ( a ) Real-time change in average traction force exerted by representative hMSCs cultured on stiff (blue), soft (red) and in situ -stiffened (soft to stiff, green) hydrogels. ( b ) Colour traction maps of representative hMSCs on stiff and soft MeHA hydrogels. The pseudocolour bar indicates the spatial traction forces, |T|, in Pa. Scale bar is 25 μm. ( c ) Time-lapse phase-contrast images and corresponding traction stress maps of a representative cell showing the real-time response to in situ stiffening (same cell). Colour map indicates the magnitude of the cellular traction stresses. Scale bar is 50 μm. ( d ) Average cellular traction force per cell area for hMSCs cultured on soft (3 kPa) and stiff (30 kPa) hydrogels for 1 day. Error bars represent s.e. ( n =20). #denotes P <0.001. ( e ) Average cellular traction plotted against corresponding cell area over a 14 h period, immediately after in situ stiffening. Each data set represents an individual cell ( n =3). Linear fit is plotted as solid line (slope=0.046). Full size image Long-term hMSC response to temporal stiffening To investigate the effect of substrate stiffening and time of stiffening on stem cell lineage commitment, hMSCs were cultured on soft substrates in bipotential differentiation medium supportive of both osteogenic (bone) and adipogenic (fat) differentiation for 14 days, during which the substrate was stiffened at different times, including days 1 (dynamic (Dyn) D1), 3 (Dyn D3) and 7 (Dyn D7; Fig. 4a , Supplementary Fig. S9 ). Control experiments were also performed, in which the cells were cultured on static soft and static stiff substrates. During the 14 days of culture, there were no statistical differences in the hydrogel elastic moduli for static soft, static stiff and stiffened substrates between any of the time points, and there were no statistical differences between the static stiff and stiffened substrates at any time point ( Supplementary Fig. S9 ). After 14 days of culture in bipotential differentiation medium, hMSCs cultured on the stiff substrates (static) primarily stained positive for alkaline phosphatase (ALP) and osteocalcin (OC), markers for osteogenic differentiation, whereas for soft substrates (static), hMSCs primarily stained positive for oil red O and fatty acid binding protein 4 (FABP4), markers for adipogenic differentiation ( Fig. 4b,c , and Supplementary Fig. S10 ). Note that we did not observe any ALP staining for hMSCs cultured entirely on soft substrates or any lipid droplets for hMSCs cultured entirely on stiff substrates. Moreover, hMSCs cultured in growth media stained negative for ALP, OC, oil red O and FABP4, independent of the substrate condition. hMSC proliferation decreased when gels were stiffened at later times ( Supplementary Fig. S9 ). Likewise, the expression of adipogenic genes was higher on the static soft substrates and the expression of osteogenic genes was higher on the static stiff substrates ( Fig. 4d ). These results confirm previous studies, in which the ability of a cell to generate tension and spread on two-dimensional substrates leads to osteogenic differentiation, whereas rounded cells primarily undergo adipogenic differentiation [40] , [41] , [42] , [43] . However, there has been no previous work to investigate hMSC differentiation responses to changing substrate stiffness. For substrates where the stiffness changes with time, the extent of staining and gene expression for osteogenic markers by hMSCs was greater for the substrates that were stiffened at earlier times, whereas the extent of staining and gene expression for adipogenic markers was greater for the substrates that were stiffened at later times ( Fig. 4b–d ). 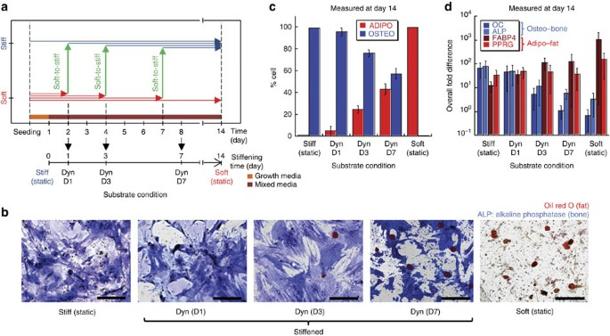Figure 4: Temporal stiffeningin situregulates hMSC differentiation. (a) Plot indicating the time line for temporal stiffening during differentiation experiments. Red and blue arrows indicate the culturing time of hMSCs on soft and stiff substrates, respectively. Green arrows indicate the time of substrate stiffening (soft to stiff). For all conditions, cells were cultured 1 day in growth media followed by 14 days in bipotential (adipo/osteo) differentiation medium (mixed media). Substrate condition is defined as static or dynamic (Dyn), and for dynamic gels stiffening time (D1, D3, D7 for 1, 3 and 7 days, respectively, of culture in mixed media before stiffening) is reported. (b) Bright-field images of hMSCs stained for ALP (osteo) and lipid droplets with oil red O (adipo) after 14 days of culture in mixed media on MeHA hydrogels stiffened at indicated days. Scale bars are 50 μm. (c) Mean percentages of hMSCs stained positive for ALP (osteo) and oil red O (adipo) as a function of stiffening time. Error bars indicate the s.d. (n=3). (d) The overall fold difference of osteogenic (OC, ALP) and adipogenic (FABP4, peroxisome proliferator-activated receptor gamma (PPRG)) gene expression obtained from RT–PCR experiments as a function of stiffening time. Error bars indicate the s.d. (n=3). Figure 4: Temporal stiffening in situ regulates hMSC differentiation. ( a ) Plot indicating the time line for temporal stiffening during differentiation experiments. Red and blue arrows indicate the culturing time of hMSCs on soft and stiff substrates, respectively. Green arrows indicate the time of substrate stiffening (soft to stiff). For all conditions, cells were cultured 1 day in growth media followed by 14 days in bipotential (adipo/osteo) differentiation medium (mixed media). Substrate condition is defined as static or dynamic (Dyn), and for dynamic gels stiffening time (D1, D3, D7 for 1, 3 and 7 days, respectively, of culture in mixed media before stiffening) is reported. ( b ) Bright-field images of hMSCs stained for ALP (osteo) and lipid droplets with oil red O (adipo) after 14 days of culture in mixed media on MeHA hydrogels stiffened at indicated days. Scale bars are 50 μm. ( c ) Mean percentages of hMSCs stained positive for ALP (osteo) and oil red O (adipo) as a function of stiffening time. Error bars indicate the s.d. ( n =3). ( d ) The overall fold difference of osteogenic (OC, ALP) and adipogenic (FABP4, peroxisome proliferator-activated receptor gamma (PPRG)) gene expression obtained from RT–PCR experiments as a function of stiffening time. Error bars indicate the s.d. ( n =3). Full size image To further explain the mixed adipogenic/osteogenic population observed for stiffened substrates, additional characterisation was performed at day 7 (in mixed media), a time point where substrate stiffening leads to near equal differentiation fates at day 14 (Dyn D7, Fig. 4c ). The cell area distribution of hMSCs on soft and stiff substrates were significantly different at this point, such that a very narrow distribution with much lower area values (60% cells with Ã~ 500 μm 2 ) were observed for hMSCs on static soft substrates (at day 7) when compared with a broader distribution with much higher area values (14% cells with Ã ~3,000 μm 2 ) for hMSCs on stiff substrates (at day 8; Figs 5a and b ). Interestingly, the distribution of cell areas of hMSCs on stiffened substrates (Dyn D7) at day 8 showed two distinct cell area populations, including a narrow cell area distribution identical to that on static soft substrates and a broader distribution at much higher values identical to that of static stiff substrates. Therefore, in contrast to the hMSC response to stiffening at day 1 (Dyn D1), where all of the cells spread and take an identical distribution to a stiff substrate 1 day after stiffening, ~42% of the cells did not spread and preserved their cell area at day 8 after stiffening at day 7. Likewise, the population that did not spread already stained positive for oil red O at this point, indicating their early differentiation towards an adipogenic lineage. The remaining ~58% of cells spread, leading to an identical cell area distribution to hMSCs on the stiff substrates, and did not stain positive for either ALP or lipid droplets. Thus, these results suggest that a population of already differentiating hMSCs were not responsive to the change in mechanical properties during the stiffening process, whereas an undifferentiated population was responsive to the change. To further confirm this result, individual hMSCs were tracked after stiffening at day 7 ( Supplementary Movies 4 ). Adipogenic cells that showed lipid droplet formation remained rounded ( Fig. 5c ), whereas undifferentiated rounded cells spread 1 day after stiffening ( Fig. 5d ), leading to a mixed population of adipogenic and undifferentiated cells at day 8 ( Fig. 5e ). 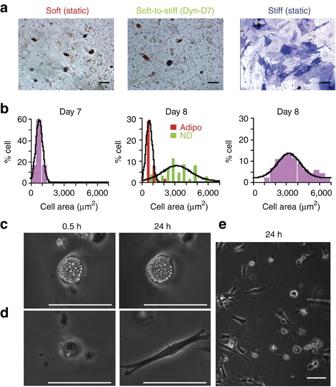Figure 5: hMSC response to stiffening determined by differentiation state. (a) Bright-field images of hMSCs stained for ALP and lipid droplets after 7 days of culture on soft and stiff hydrogels, and 8 days of culture on hydrogels stiffened at day 7. (b) Corresponding cell area distributions for hMSCs in (a). For hMSCs on stiffened hydrogels, area distributions are plotted in two populations, including adipogenic cells (adipo) that are stained positive for oil red O and non-differentiated cells (ND) that are not stained positive for either alkaline phosphatase or oil red O. (c,d) Phase-contrast images of representative hMSCs at 0.5 and 24 h after stiffening at day 7. (e) Phase-contrast image showing the mixed population of hMSCs 24 h after stiffening at day 7. All scale bars are 100 μm. Figure 5: hMSC response to stiffening determined by differentiation state. ( a ) Bright-field images of hMSCs stained for ALP and lipid droplets after 7 days of culture on soft and stiff hydrogels, and 8 days of culture on hydrogels stiffened at day 7. ( b ) Corresponding cell area distributions for hMSCs in ( a ). For hMSCs on stiffened hydrogels, area distributions are plotted in two populations, including adipogenic cells (adipo) that are stained positive for oil red O and non-differentiated cells (ND) that are not stained positive for either alkaline phosphatase or oil red O. ( c , d ) Phase-contrast images of representative hMSCs at 0.5 and 24 h after stiffening at day 7. ( e ) Phase-contrast image showing the mixed population of hMSCs 24 h after stiffening at day 7. All scale bars are 100 μm. Full size image To investigate the involvement of the actin cytoskeleton in dynamic stiffening, hMSCs were treated with cytochalasin D, an actin-disrupting agent, which prevented cellular spreading in response to stiffening ( Fig. 6a , Supplementary Fig. S11 ). We observed a significant increase in adipogenesis and no osteogenesis for hMSCs cultured on soft substrates for 7 days, followed by 7 days of culture in cytochalasin D-treated mixed media ( Fig. 6b ) compared with the observed mixed population of adipogenic/osteogenic hMSCs cultured in the absence of cytochalasin D ( Fig. 4c ). We also inhibited myosin-generated cytoskeletal tension by treating hMSCs with Y-27632, an inhibitor of Rho kinase that is involved in myosin activation, and blebbistatin, a myosin II inhibitor. In the presence of Y-27632, undifferentiated cells responded to stiffening at day 7 and become morphologically similar to untreated cells at day 8, but did not stain positive for ALP at day 14 ( Fig. 6b ). Similarly, blebbistatin treatment significantly reduced the osteogenic differentiation of uncommitted cells, although the cells also were morphologically similar to untreated cells at day 8 ( Fig. 6a ). These results were in agreement with the reported hMSC response on stiff substrates in the presence of these disrupting agents [42] . 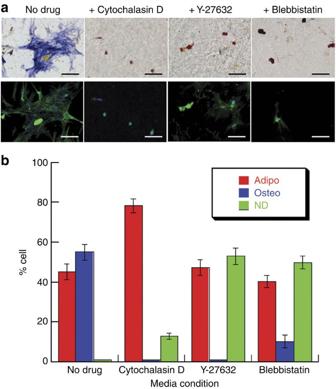Figure 6: hMSC response to stiffening and corresponding differentiation state change with cytoskeletal tension and signalling. (a) Bright-field images of hMSCs stained for ALP and lipid droplets (LD) after 14 days of culture in mixed media on dynamic substrates, which were stiffened at day 7 (Dyn-D7). The subgroups refer to the treatment condition of the mixed media following stiffening at day 7. Mixed media with cytochalasin D (blocks actin polymerisation), Y-27632 (blocks Rho kinase (ROCK) signalling), blebbistatin (blocks myosin contractility), or without any treatment (no drug) during the remaining 7-day culture period after stiffening. Scale bars are 100 μm. (b) Corresponding cell percentage that are stained positive for LD (adipo), ALP (osteo) and non-differentiated cells (ND), that are not stained positive for either ALP or LD, with or without treatment. Error bars indicate the s.d. (n=3). Figure 6: hMSC response to stiffening and corresponding differentiation state change with cytoskeletal tension and signalling. ( a ) Bright-field images of hMSCs stained for ALP and lipid droplets (LD) after 14 days of culture in mixed media on dynamic substrates, which were stiffened at day 7 (Dyn-D7). The subgroups refer to the treatment condition of the mixed media following stiffening at day 7. Mixed media with cytochalasin D (blocks actin polymerisation), Y-27632 (blocks Rho kinase (ROCK) signalling), blebbistatin (blocks myosin contractility), or without any treatment (no drug) during the remaining 7-day culture period after stiffening. Scale bars are 100 μm. ( b ) Corresponding cell percentage that are stained positive for LD (adipo), ALP (osteo) and non-differentiated cells (ND), that are not stained positive for either ALP or LD, with or without treatment. Error bars indicate the s.d. ( n =3). Full size image We developed a material platform that enables temporal matrix stiffening in the presence of cells, which mimics the dynamic nature of many biological processes, such as tissue development, wound healing and disease formation. Our objective was a system where hydrogel stiffening is obtained rapidly and in a well-controlled and -defined manner, with structural and mechanical homogeneity and long-term stability. This was achieved by exploiting two methods of crosslinking through the same reactive group (that is, MeHA, where initial gelation is obtained via an addition reaction, and the gel is stiffened by secondary crosslinking through a light-mediated radical polymerisation). This technique can also be used to apply temporal stiffening spatially, as light is used as the material trigger and can be applied to any reactive polymer that contains groups that can undergo both types of polymerisation. However, this process only leads to increased stiffening (as observed in biological events such as fibrosis) and it is not possible to decrease mechanics with cells present due to irreversible crosslinking. Additionally, the stiffness changes occur quite rapidly in this system and do not directly mimic the typical native stiffening behaviour of biological events such as tissue development and disease formation. For instance, maturation of myocardium (~10 kPa) from mesoderm (<0.5 kPa) is reported to require up to 2 weeks in chicken [44] , [45] . Similarly, fibrotic stiffening of the heart muscle post-heart attack may take several weeks [46] , [47] . However, it is possible to control the rate of stiffening in our system by applying multiple exposures, during which the rate of stiffness change can be controlled by time between exposures, and the stiffness in each step can be controlled by the exposure time ( Supplementary Fig. S2 ). To demonstrate the utility of our system, we investigated the short- (hours) and long-term (days to weeks) cell response to dynamic stiffening (from ~3 to 30 kPa as a model system). An increase in mean cell area from ~400 to ~1500 μm 2 occurred within 4 h immediately on stiffened substrates, whereas little change in cell area was observed on static soft (~400 μm 2 ) and stiff (~1500 μm 2 ) substrates during this period. Likewise, the average traction of hMSCs increased significantly from ~1 to 10 kPa within 4 h and linearly correlated with the increase in cell area. One important area of investigation is the behaviour of stem cells in their microenvironment, and until now, most of these studies were focussed on static tissue culture plates or hydrogels. With this new system, we sought to understand how hMSCs behave in a material microenvironment where the biophysical properties change during the period of differentiation. A model system was utilised, in which the hMSCs were cultured in a mixed soluble media that permits both osteogenic (bone) and adipogenic (fat) differentiation, and cells were cultured for 14 days, with substrate stiffening after 1, 3 and 7 days. Our results show that hMSCs differentiate into mixed populations based on how long they are cultured on a substrate of a specific stiffness, such that adipogenic differentiation is favoured the longer the cell is on the softer substrate (stiffening at later times), whereas osteogenic differentiation increases the longer the cell is on the stiffer substrate (stiffening at early times). Interestingly, a mixed adipogenic/osteogenic population was observed for dynamic substrates stiffened at day 7 during 14 days of culture in mixed differentiation media. In fact, two distinct cell populations were observed with respect to cell area at day 8 (1 day after stiffening) on the same dynamic substrates stiffened at day 7, including a narrow cell area distribution identical to that on the soft substrates before stiffening, and a broader distribution at much higher values identical to that of the static stiff substrates. Further investigation revealed that the hMSC population that remained rounded after stiffening stained positive for oil red O at this point, indicating their early differentiation towards an adipogenic lineage. Moreover, hMSCs that had spread morphology at day 8 did not stain positive for either ALP or lipid droplets; however, there was positive staining for ALP at day 14, which indicated that this spread-cell population differentiated towards an osteogenic lineage when enough time was provided. Thus, these results suggest that a population of already differentiating hMSCs were not responsive to the change in mechanical properties during the stiffening process, whereas an undifferentiated population was responsive to the change. In this work, the bipotential mixed differentiation media was needed for differentiation of hMSCs, independent of the substrate stiffness. Our work shows that there is an inherent heterogeneity to the hMSC population, even though the starting hMSCs exhibited high surface expression for mesenchymal markers (>90%) and were negative for hematopoietic markers (<10%) [48] , [49] , [50] . Thus, we believe there was epigenetic heterogeneity to the cells, which led to differences in the rate of differentiation on the hydrogel substrates, leading to differential populations based on the timing of substrate stiffening, as committed cells did not respond to the mechanical changes. Finally, by eliminating the uncommitted hMSC response to stiffening at day 7 by blocking actin polymerisation, we observed a significant increase in adipogenesis and limited osteogenesis at day 14, confirming the mechanical effect of the stiffening process. When myosin activation or Rho kinase pathway were blocked after stiffening at day 7, although the undifferentiated cell morphology was similar to that of at day 8, these cells stained primarily negative for ALP, leading to a mixed population of primarily adipogenic and undifferentiated cells. It is clear that temporal changes of substrate properties has been overlooked in most in vitro cell culture systems, despite the importance of changing cues during tissue development and healing. The results here indicate the importance of the timing of substrate stiffening on hMSC behaviour and the differentiation state of the cell at the time of stiffening. These findings clearly illustrate an example where the sequential crosslinking technique is a powerful tool to investigate dynamic changes in biological processes, an approach that may be useful to investigate tissue development, wound healing and disease progression. MeHA synthesis MeHA was synthesised following a previously described procedure [51] . Briefly, sodium hyaluronate (Lifecore, 59 kDa) was dissolved in deionised water (1 wt%) and reacted with MA (2.4 ml MA per gram of HA) at pH 8.0 on ice for 8 h, followed by overnight incubation (at 4 °C), and further reaction with MA (1.2 ml MA per gram of HA) at pH 8.0 on ice for 4 h. The macromer solution was purified via dialysis in deionised water (SpectraPor, molecular weight cutoff, 6–8 kDa) at 4 °C for 3 days and lyophilised. 1 H NMR (Bruker) was used to confirm modification (~100%) of the hydroxyl groups on the HA backbone. Fabrication of MeHA substrates for cell culture MeHA substrates (soft, E ~3 kPa) were fabricated using Michael-type addition polymerisation, during which crosslinking occurs via introduction of DTT (20%, except for variable DTT investigation) to a 3 wt% solution of MeHA in PBS buffer containing 0.2 M triethanolamine (at pH 10, except for variable pH studies) and 0.05 wt% I2959 (Ciba). MeHA solution (110 μl) was pipetted into a poly(dimethylsiloxane) mold (Sylgard 184 ® Silicone Elastomer Kit, Dow Corning, ~200 μm thick) and covered with a methacrylated glass slide (prepared as in Guvendiren et al ., [52] ) and incubated for 1 h at room temperature to obtain a crosslinked substrate (addition-only). To fabricate stiff ( E ~30 kPa) substrates, soft substrates were exposed to ultraviolet light (10 mW cm −2 ) for 2 min after incubation in media containing I2959 photoinitiator (0.05 wt%). An oligopeptide GCGYGRGDSPG (GenScript) was added into the MeHA solution before DTT addition, and reacted for 30 min to couple RGD adhesion moiety into the MeHA, such that the final concentration of RGD was 1 mM. To study the effect of RGD concentration on cellular behaviour, MeHA substrates with various RGD concentrations (0, 0.5, 1, 1.5, 2 mM) were also prepared. For cell studies, MeHA substrates were incubated in sterile PBS overnight and washed with sterile PBS. MeHA substrates were then sterilised under a germicidal lamp for 2 h in sterile PBS and incubated in growth media for 30 min before cell seeding. For time-lapse cell imaging and TFM, MeHA substrates were crosslinked on larger coverslips (45×50 mM) and sealed at the bottom of a culture chamber. For TFM experiments, MeHA substrates were embedded with 1-μm diameter fluorescent microspheres (FluoSpheres ® , Invitrogen, Molecular Probes). These substrates were crosslinked top surface facing down, allowing beads to segregate at the top surface. In this case, the pH of MeHA solution was set to 8 to slow crosslinking, giving beads enough time to segregate before gelation, while keeping the substrate mechanics identical to substrates obtained at pH 10. We would like to note that as hydrogel substrates were attached to a glass slide, they can only swell (or deswell) perpendicular to the substrate surface eliminating the potentially significant strains on the gels in the case of free swelling gels. The thickness of the initially formed hydrogel substrates (200 μm thick) equilibrated to 250 μm when immersed in PBS and culture media, and deswell to become 200 μm immediately after stiffening. Characterisation of crosslinking kinetics and substrate mechanics Dynamic oscillatory time sweeps were performed using an AR2000ex rheometer (TA Instruments) with an ultraviolet light-guide accessory (SmartSwap™, TA Instruments) connected to an ultraviolet light source (Exfo Omnicure S2000). Storage (G′) and loss moduli (G′′) with time were monitored under 0.5% strain and 1 Hz, using a cone and plate geometry (1°, 20-mm diameter) at 25 °C, and a solvent trap was used to prevent sample evaporation. For sequential crosslinking experiments, I2959 was added into the MeHA solution before loading. After initial gelation via addition-only polymerisation, the sample was exposed to ultraviolet light (10 mW cm −2 , 365 nm). Mechanical properties of the MeHA substrates were measured by atomic force microscopy, as described previously [52] . Cell culture and reagents The hMSCs (Lonza Corp.) were expanded in growth medium (α-MEM, 10% fetal bovine serum, 1% L -glutamine and 1% penicillin streptomycin). The hMSCs were reported to be positive for mesenchymal surface markers (>90% CD105, CD166, CD29 and CD44) and negative for hematopoietic markers (<10% CD14, CD34 and CD45). To ensure the undifferentiated state of hMSCs, we used early passage cells (passage 3) that are previously reported to maintain these same levels of surface markers [48] , [49] , [50] . In this study, hMSCs at passage 3 were seeded onto MeHA substrates at 5×10 3 cells per cm 2 . For differentiation studies, after 1 day of incubation in growth medium, cells were maintained in bipotential differentiation medium consisting of 1/1 adipogenic/osteogenic induction media (R&D Systems Inc.), supplemented with 1% penicillin streptomycin, for up to 14 days (refreshing media every 3 days). Proliferation was measured by comparing the number of cell nuclei before (after 1 day culture in growth media) and after 14 days of mixed media culture. In situ stiffening during culture The hMSCs were cultured on soft MeHA substrates in growth or bipotential differentiation media in a six-well plate. MeHA substrates were stiffened at a user-defined time during the hMSC culture via radical polymerisation by ultraviolet light exposure (10 mW cm −2 , 365 nm). Before substrate stiffening, the media (3 ml per well) was replaced with I2959-containing media (0.05 wt%) and incubated for 30 min at 37 °C, followed by exposure to ultraviolet light for 2 min. Immediately after exposure, the substrates were washed three times with fresh media. No loss of cell viability or DNA damage was observed under these conditions. Cell staining Cells were fixed in 4% formalin for 10 min. For morphology studies, hMSCs were stained for F-actin with TRITC-phalloidin and for nuclei with DAPI (Invitrogen), after extracting the soluble component (0.25% Triton) and blocking the non-specific binding sites (with 3% bovine serum albumin and 0.1% Tween-20 in PBS). For differentiation studies, cells were stained for ALP with Fast Blue RR/napthol solution, lipid droplets using 3 mg ml −1 oil red O in 60% isopropanol, and nuclei with DAPI. Phase-contrast and fluorescent images of the cells were captured on an Olympus BX51 microscope. For cell area measurements of stained hMSCs, fluorescent images of cells were taken from the substrate surface. NIH ImageJ was used to measure the cell area for each hMSC. The data was binned and histograms were plotted with Gaussian fits using KaleidaGraph ® . For immunostaining, fixed cells were subsequently permeabilised and blocked (0.1% triton X-100, 1% bovine serum albumin and 10% horse serum in PBS) at room temperature for 45 min. Cells were then incubated with primary antibody (FABP, OC, p53 (R&D), or vinculin (Sigma)) overnight at 4 °C, followed by appropriate secondary antibody (Invitrogen) at room temperature for 2 h. Cell viability was assessed by using a live/dead staining kit (Molecular Probes) and alamar blue assay (Invitrogen). Time-lapse microscopy Time-lapse images of individual cells (40× objective) or groups of cells (10× and 20× objective) were captured at 30-min intervals for a minimum of 16 h for each substrate group, using a Photometric Cool Snap HQ camera (Roper Scientific) connected to a Nikon Inverted Eclipse TE300 microscope equipped with a high-speed motorised XY stage, enabling programming of automated image collection. The microscope system was confined in a custom-made environmental chamber at 37 °C and 5% CO 2 . Traction-force microscopy Forces exerted by hMSCs on MeHA substrates were measured via TFM, based on deformations in the substrate relative to the same substrate when relaxed, using a method developed by Dembo and Wang [53] . In this method, surface traction vectors generated by the cells on the underlying substrate were quantified by measuring embedded bead displacements and using known substrate properties (thickness, modulus) with custom-written software [53] . For this purpose, phase-contrast and corresponding fluorescent bead images were collected simultaneously using the microscope system described above. At the end of each experiment, fluorescent images of the beads in the relaxed substrate were captured after the cells were completely released from the substrate, using trypsin–EDTA. TFM microscopy was performed for hMSCs, on soft and stiff substrates in growth media, at day 1 and 2 and for hMSCs on stiffened substrates at day 2. Time-lapse phase-contrast and fluorescent images were also collected on soft, stiff and stiffened substrates at 30-min intervals for 16 h. For stiffened substrates, image collection began immediately after light exposure. Real-time PCR After 14 days of culture in bipotential differentiation medium, MeHA substrates, static and dynamic (stiffened), were removed from the wells and digested in 1 ml Trizol reagent (Invitrogen). At least four substrates were sampled and digested together for each condition, repeated three times. PCR was conducted on a real-time PCR machine (RT–PCR 7,300, Applied Biosystems) using primers and Taqman probes (Applied Biosystems) specific for glyceraldehyde 3-phosphate dehydrogenase ( GAPDH , housekeeping gene), ALP, OC, FABP4 and peroxisome proliferator-activated receptor gamma ( PPRG ). Gene expression relative to hMSCs at the time of seeding was determined using the ΔΔCt method. How to cite this article: Guvendiren, M. et al . Stiffening hydrogels to probe short- and long-term cellular responses to dynamic mechanics. Nat. Commun. 3:792 doi: 10.1038/ncomms1792 (2012).